Organization of the mitochondrial translation machinery studiedin situby cryoelectron tomography Whereas the structure and function of cytosolic ribosomes have been studied in great detail, we know surprisingly little about the structural basis of mitochondrial protein synthesis. Here we used cryoelectron tomography and subtomogram analysis to visualize mitoribosomes in isolated yeast mitochondria, avoiding perturbations during ribosomal purification. Most mitoribosomes reside in immediate proximity to the inner mitochondrial membrane, in line with their specialization in the synthesis of hydrophobic membrane proteins. The subtomogram average of membrane-associated mitoribosomes reveals two distinct membrane contact sites, formed by the 21S rRNA expansion segment 96-ES1 and the inner membrane protein Mba1. On the basis of our data, we further hypothesize that Mba1 is not just a passive mitoribosome receptor on the inner membrane, but that it spatially aligns mitoribosomes with the membrane insertion machinery. This study reveals detailed insights into the supramolecular organization of the mitochondrial translation machinery and its association with the inner membrane in translation-competent mitochondria. Mitochondria are essential organelles of eukaryotic cells, which produce ATP by aerobic respiration. They maintained their own translation machinery, mostly for the synthesis of a few highly hydrophobic membrane proteins that form the central reaction centres of the enzymes of the respiratory chain and the ATP synthase [1] . Mitochondrial translation products are co-translationally integrated into the inner membrane in a reaction that depends on two factors in yeast: (1) Oxa1, the homologue of the bacterial YidC, serves as an integrase that inserts its client proteins into the inner membrane [2] , [3] , [4] , [5] . (2) Mba1 (mammalian homologue: Mrpl45 or mL45) cooperates with Oxa1 in the membrane recruitment of mitoribosomes [6] , [7] . Biochemical studies suggest that the mitoribosome remains associated to the inner membrane even in mutants lacking both Oxa1 and Mba1, indicating the presence of additional, so far unidentified membrane tethers [7] , [8] . Only very recently, high-resolution structures for the large subunit of the mammalian and yeast mitoribosome [9] , [10] and the small subunit of the mammalian mitoribosome [11] were published. Since the mitoribosomes used in these single particle cryo-electron microscopy (cryo-EM) experiments were recovered from salt-washed detergent extracts, membrane-binding sites remained hypothetical. On the basis of earlier cryo-EM studies it was speculated that the mitoribosome might be partially embedded into the lipid bilayer [12] , whereas the recent high-resolution studies led to the hypotheses that the mitoribosome resides in the mitochondrial matrix and contacts the inner membrane either via a mitoribosome-specific protuberance of the large subunit [9] or the peptide exit associated protein Mrpl45 (ref. 10 ). To avoid perturbations during ribosomal purification, we used an alternative approach that does not require the purification of ribosomal particles and allows studying the membrane association of mitoribosomes in situ . Cryoelectron tomography (CET) is an excellent method for studying the structure of large molecules in their natural context [13] , in particular ribosomal structures and their supramolecular assembly [14] , [15] , [16] . Using this approach, we analysed mitoribosome structure and distribution in purified translation-competent mitochondria revealing detailed insights into the organization of the mitochondrial translation machinery and its association with the inner membrane. Yeast mitoribosomes are in proximity to the inner membrane Mitochondria were isolated from wild-type yeast cells and the functionality of their translation and membrane insertion machinery was verified by in organello translation, indicating synthesis and processing of all eight proteins encoded by the mitochondrial genome ( Fig. 1a ). In tomograms of those mitochondria, mitoribosomes and ATP synthases are the most prominent macromolecular complexes and are readily discernable in the mitochondrial matrix ( Fig. 1b ). To analyse the spatial distribution of mitoribosomes in mitochondria, candidate particles were located by a six-dimensional cross-correlation search (‘template matching’) against a single particle cryo-EM reconstruction of the yeast 73S mitoribosome [9] . Features coinciding with cross-correlation peaks were visually inspected to identify true positive matches. For three representative tomograms, we manually traced the mitochondrial inner membrane ( Supplementary Fig. 1 ) and determined the shortest Euclidean distance from all mitoribosome positions to the membrane in these three tomograms. According to the distribution of mitoribosome-membrane distances ( Fig. 1c ), most mitoribosomes reside in immediate proximity of the inner membrane, with a preferred distance of 17 nm between the membrane and their positional coordinates. Assuming an approximate radius of 13–14 nm for the mitoribosome, this corresponds to a preferred distance of 3–4 nm between the ribosomal surface and the membrane. This finding strongly supports the notion that in yeast the vast majority of mitoribosomes is tethered to the inner mitochondrial membrane. 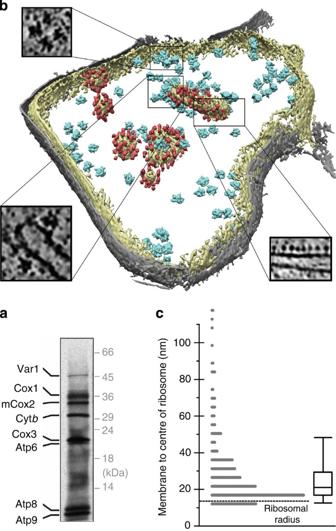Figure 1: Distribution of mitoribosomes in translation-competent yeast mitochondria. (a) Isolated mitochondria were labelled for 10 min with radioactive methionine and synthesized proteins were visualized by SDS–PAGE and autoradiography. The synthesized translation products are indicated. mCox2 indicates mature processed Cox2. (b) Rendered and segmented version of a tomogram depicting the outer (grey) and inner mitochondrial membrane (yellow) detected mitoribosomes visualized by the template (blue) and a subset of ATP synthases (red). Mitoribosomes and ATP synthases can be readily discerned in mildly Gaussian-filtered (1.5 nm width) slices of the tomogram (boxed areas). (c) Distribution of shortest distances between the centre of mass of detected mitoribosomes and the inner mitochondrial membrane represented as histogram and box-whisker plot for 478 mitoribosomes from three tomograms. The box includes the median, upper and lower quartiles of the distribution. Box whiskers include 80% of the data to indicate variability outside the upper and lower quartiles. The dashed line corresponds to the approximate radius of a mitoribosome (14 nm). Figure 1: Distribution of mitoribosomes in translation-competent yeast mitochondria. ( a ) Isolated mitochondria were labelled for 10 min with radioactive methionine and synthesized proteins were visualized by SDS–PAGE and autoradiography. The synthesized translation products are indicated. mCox2 indicates mature processed Cox2. ( b ) Rendered and segmented version of a tomogram depicting the outer (grey) and inner mitochondrial membrane (yellow) detected mitoribosomes visualized by the template (blue) and a subset of ATP synthases (red). Mitoribosomes and ATP synthases can be readily discerned in mildly Gaussian-filtered (1.5 nm width) slices of the tomogram (boxed areas). ( c ) Distribution of shortest distances between the centre of mass of detected mitoribosomes and the inner mitochondrial membrane represented as histogram and box-whisker plot for 478 mitoribosomes from three tomograms. The box includes the median, upper and lower quartiles of the distribution. Box whiskers include 80% of the data to indicate variability outside the upper and lower quartiles. The dashed line corresponds to the approximate radius of a mitoribosome (14 nm). Full size image Mitoribosomes show a pronounced short-range order In our tomograms, mitoribosomes are typically organized in clusters on the inner mitochondrial membrane ( Fig. 1b ), suggesting the presence of membrane-bound polyribosomes. Both, membrane- [15] and non-membrane-bound [16] , [17] cytosolic polyribosomes typically show a specific close-range order between adjacent ribosomes, resulting in a characteristic architecture of the polyribosome. In order to analyse the three-dimensional (3D) arrangement of membrane-bound mitoribosomes, we pursued a strategy similar to our analysis of ribosome arrangements on the ER membrane [15] . First, we extracted a list of pairwise mitoribosome arrangements from the positional coordinates, which was filtered to arrangements complying with a preferred Euclidean interparticle distance (20–40 nm, Supplementary Fig. 2a ) and membrane inclination (0–50°, Supplementary Fig. 2b ). For a detailed analysis, we chose a coordinate system, in which the mitochondrial inner membrane (as observed in the subtomogram average described below) corresponds to the paper plane. In this coordinate system, we defined two angles describing the relative position ( α ) and relative orientation ( β ) of adjacent mitoribosomes ( Fig. 2a ). Plotting of α against β yielded two highly populated classes (I and II) on a scarcely populated background ( Fig. 2b ). Visualization of these two arrangements by replicates of the template structure, positioned according to averaged coordinates and rotations of the classes, indicates that both classes represent the same linear arrangement of mitoribosomes, corresponding to the left and the right neighbours in the polyribosome, respectively. This arrangement of mitoribosomes results in a slightly curved architecture of the polyribosome with a smooth pathway of modelled polysomal mRNA interconnecting neighbouring mitoribosomes ( Fig. 2c ). Within the two classes, α and β are strongly correlated. To visualize the consequences of this correlation of relative neighbour position and orientation on polysome architecture, we subdivided class I into three equally populated subclasses (I–I to I–III) according to the relative position of adjacent mitoribosomes ( Fig. 2d ). In the resulting arrangements ( Fig. 2e ), we observed that the local correlation of relative positions and orientations within the class causes a radial movement of the neighbour around the mitoribosome under scrutiny, likely guided by their physical interaction via the polysomal mRNA. 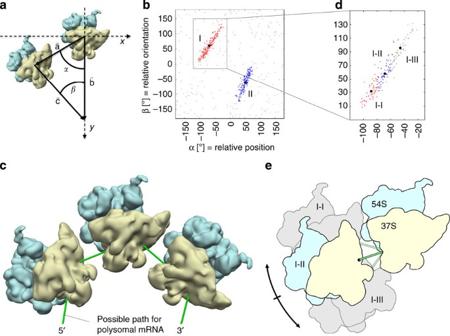Figure 2: Three-dimensional arrangement of mitoribosomes in membrane-bound polyribosomes. (a) For the analysis of the 3D distribution of mitoribosomes, two angles were defined: the angleαbetween theyaxis of the mitoribosome under scrutiny and the centre-to-centre vectorof another mitoribosome describes their relative positions, while the angleβbetween the vectorsandof the two mitoribosomes captures their relative orientation. (b) The plot ofαagainstβand subsequent clustering of the data set (730 pairwise mitoribosome arrangements) reveals two highly populated classes I and II that represent the left and right neighbour in the same 3D arrangement of mitoribosomes. (c) Preferred 3D arrangement of membrane-bound mitoribosomes, visualized by replicates of the template structure, looking down on the inner membrane. The shortest path between mRNA entry and exit sites of adjacent mitoribosomes was indicated (green) to visualize a possible pathway for polysomal mRNA. (d) Class I frombwas further subdivided into three equally populated clusters (I–I to I–III) according to the relative position of adjacent mitoribosomes. (e) Schematic representation of the ribosomal arrangements represented by classes I–I to I–III and the modelled pathways of polysomal mRNA. Figure 2: Three-dimensional arrangement of mitoribosomes in membrane-bound polyribosomes. ( a ) For the analysis of the 3D distribution of mitoribosomes, two angles were defined: the angle α between the y axis of the mitoribosome under scrutiny and the centre-to-centre vector of another mitoribosome describes their relative positions, while the angle β between the vectors and of the two mitoribosomes captures their relative orientation. ( b ) The plot of α against β and subsequent clustering of the data set (730 pairwise mitoribosome arrangements) reveals two highly populated classes I and II that represent the left and right neighbour in the same 3D arrangement of mitoribosomes. ( c ) Preferred 3D arrangement of membrane-bound mitoribosomes, visualized by replicates of the template structure, looking down on the inner membrane. The shortest path between mRNA entry and exit sites of adjacent mitoribosomes was indicated (green) to visualize a possible pathway for polysomal mRNA. ( d ) Class I from b was further subdivided into three equally populated clusters (I–I to I–III) according to the relative position of adjacent mitoribosomes. ( e ) Schematic representation of the ribosomal arrangements represented by classes I–I to I–III and the modelled pathways of polysomal mRNA. Full size image Mitoribosomes bind to the inner membrane in a defined way In order to obtain detailed insights into the association of mitoribosomes with the inner membrane, subtomograms depicting mitoribosomes were individually reconstructed at full resolution, iteratively aligned and sorted by two consecutive unsupervised classification rounds. In the first sorting round, classification of 1,674 initial subtomograms from 12 tomograms was focused on the 37S subunit to separate 73S mitoribosomes from small populations of 54S ribosomal subunits (7%) and 73S mitoribosomes with a hyper-rotated 37S subunit (3%; Fig. 3a ). In the second round of classification, focused on the membrane region and the 54S subunit, subtomograms with clearly visible density for the inner mitochondrial membrane were enriched ( Fig. 3b ). Iterative re-alignment of the remaining 900 subtomograms yielded a structure of the 73S mitoribosome bound to the mitochondrial inner membrane ( Fig. 4a ) with an overall resolution of 28 Å ( Fig. 5a ). The local resolution of the map varies according to position, with an approximate value of 22 Å at the core of the mitoribosome and ~30 Å in the membrane region ( Fig. 5b ). Consistently, Fourier shell correlation between a cryo-EM single particle structure of the 73S yeast mitoribosome [9] and the subtomogram average indicates a resolution of 23 Å for the ribosome part of the subtomogram average ( Fig. 5a ). The atomic model for the yeast 54S subunit [9] (PDB 1VW3, 1VW4) derived from this single particle structure shows an excellent rigid body fit into the 54S density of the subtomogram average ( Fig. 4b ). Consistent with previous cryo-EM studies [9] , [10] , [18] , the mitoribosome depicted in our subtomogram average is considerably larger than its bacterial counterpart, matching the dimensions of cytosolic 80S ribosomes ( Supplementary Fig. 3 ). Notably, a ribosome-associated density resolved in the subtomogram average close to the mRNA exit site on the 37S subunit ( Supplementary Fig. 4a ) coincides with the expected path of polysomal mRNA ( Supplementary Fig. 4b ) in the preferred arrangement described in Fig. 2c . The biochemical nature of this density is unclear, as similar structures were not present for polyribosomes of the bacterial or eukaryotic cytosol [15] , [16] , [17] . Despite its specialization on the translation of a small number of very hydrophobic membrane proteins, the yeast mitoribosome is by no means embedded in the inner membrane, as previously speculated for the mammalian mitoribosome [12] . On the contrary, the distance between the inner mitochondrial membrane and the canonical peptide exit site on the mitoribosome even exceeds that observed between eukaryotic ribosomes and the ER membrane during co-translational protein translocation ( Supplementary Fig. 5 ) [14] . 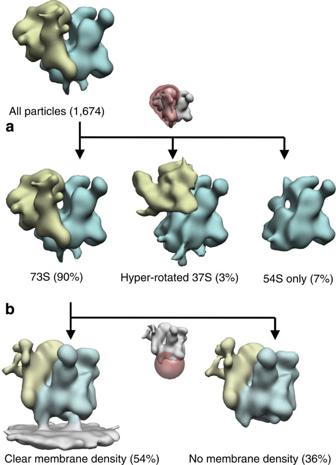Figure 3: Classification of subtomograms from wild-type mitochondria. (a) In a first round, classification was focused on the 37S subunit of the mitoribosome (classification mask depicted in red) and separated 73S mitoribosomes from 54S subunits and mitoribosomes with a hyper-rotated 37S subunit. (b) In a second round, classification was focused on the membrane and parts of the 54S subunit (classification mask depicted in red) and enriched subtomograms with clear density for the inner mitochondrial membrane. Absence of the membrane density is mostly due to orientations of particles that do not allow resolving the membrane as a consequence of the ‘missing wedge effect’ in CET. Class abundance is given as percentage of all particles. For classification round 1, the membrane region of the subtomogram average is not shown. Figure 3: Classification of subtomograms from wild-type mitochondria. ( a ) In a first round, classification was focused on the 37S subunit of the mitoribosome (classification mask depicted in red) and separated 73S mitoribosomes from 54S subunits and mitoribosomes with a hyper-rotated 37S subunit. ( b ) In a second round, classification was focused on the membrane and parts of the 54S subunit (classification mask depicted in red) and enriched subtomograms with clear density for the inner mitochondrial membrane. Absence of the membrane density is mostly due to orientations of particles that do not allow resolving the membrane as a consequence of the ‘missing wedge effect’ in CET. Class abundance is given as percentage of all particles. For classification round 1, the membrane region of the subtomogram average is not shown. 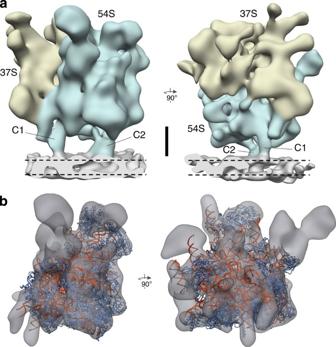Figure 4: Structure of the membrane-bound mitoribosome. (a) Subtomogram average filtered to 28 Å resolution. The 54S (blue) and 37S (yellow) subunits, the inner mitochondrial membrane (grey) and two distinct contact sites between the mitoribosome and the membrane (C1 and C2) are resolved. Dashed lines indicate the two leaflets of the membrane bilayer. The scale bar corresponds to 5 nm. (b) Atomic model of the 54S subunit (modelled proteins blue, modelled rRNA orange, PDB 1VW3, 1VW4) fitted into the 54S density of the subtomogram average (transparent grey). Some flexible parts of the 54S subunit are not included in the atomic model. Full size image Figure 4: Structure of the membrane-bound mitoribosome. ( a ) Subtomogram average filtered to 28 Å resolution. The 54S (blue) and 37S (yellow) subunits, the inner mitochondrial membrane (grey) and two distinct contact sites between the mitoribosome and the membrane (C1 and C2) are resolved. Dashed lines indicate the two leaflets of the membrane bilayer. The scale bar corresponds to 5 nm. ( b ) Atomic model of the 54S subunit (modelled proteins blue, modelled rRNA orange, PDB 1VW3, 1VW4) fitted into the 54S density of the subtomogram average (transparent grey). Some flexible parts of the 54S subunit are not included in the atomic model. 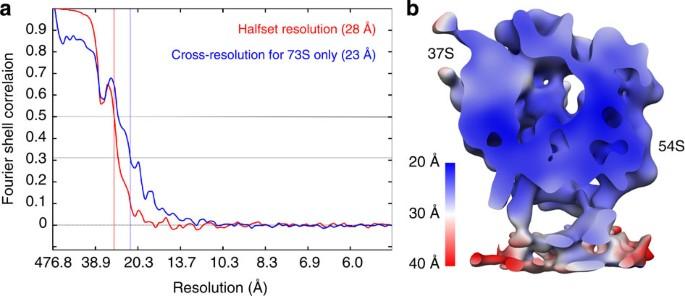Figure 5: Resolution assessment via FSC and cross-resolution. (a) The resolution of the subtomogram average was determined to 28 Å by FSC 0.5 criterion with a mask, encompassing the whole 73S mitoribosome and most of the inner mitochondrial membrane. For validation, the cross-resolution between the yeast 73S mitoribosome as determined by single particle cryo-EM9and the 73S part of the subtomogram average was determined to 23 Å (FSC 0.33 criterion). (b) Local resolution assessment of the subtomogram average with an estimated range of 22 Å at the core of the mitoribosome and ~30 Å in the mitoribosome-associated membrane region. Full size image Figure 5: Resolution assessment via FSC and cross-resolution. ( a ) The resolution of the subtomogram average was determined to 28 Å by FSC 0.5 criterion with a mask, encompassing the whole 73S mitoribosome and most of the inner mitochondrial membrane. For validation, the cross-resolution between the yeast 73S mitoribosome as determined by single particle cryo-EM [9] and the 73S part of the subtomogram average was determined to 23 Å (FSC 0.33 criterion). ( b ) Local resolution assessment of the subtomogram average with an estimated range of 22 Å at the core of the mitoribosome and ~30 Å in the mitoribosome-associated membrane region. Full size image Mitoribosomes are membrane-tethered by two contact sites The orientation and position of the mitoribosome on the inner membrane differs from a previous hypothesis on the basis of the putative involvement of a mitoribosome-specific protuberance of the large subunit in membrane tethering [9] . Instead, the mitoribosome is tethered to the inner membrane by two prominent contact sites, C1 and C2, located on opposing sites of the canonical (‘bacterial’) peptide exit tunnel ( Fig. 4a ). Superposition of the atomic model of the yeast 54S ribosomal subunit [9] (PDB 1VW3, 1VW4) to the subtomogram average reveals that one of these contacts (C1) is mediated by the 21S rRNA expansion segment 96-ES1 ( Fig. 6 ). 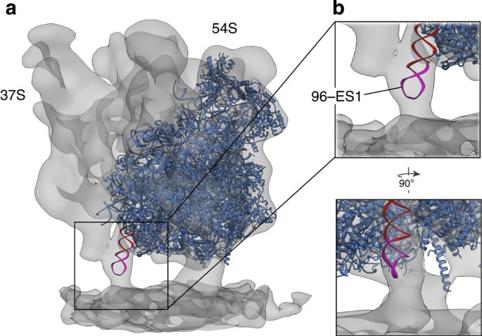Figure 6: Large subunit ribosomal RNA 96-ES1 constitutes the C1 contact site. (a) Atomic model of the 54S subunit (blue, PDB 1VW3, 1VW4) with 96-ES1 highlighted in red/magenta fitted into the subtomogram average (transparent grey) as a rigid body. Twenty residues of 96-ES1 (magenta) were not included in the original model and were extended using the tip of a random rRNA ES. (b) Zoomed views of the boxed area inashowing colocalization of 96-ES1 and the C1 contact site in more detail. Figure 6: Large subunit ribosomal RNA 96-ES1 constitutes the C1 contact site. ( a ) Atomic model of the 54S subunit (blue, PDB 1VW3, 1VW4) with 96-ES1 highlighted in red/magenta fitted into the subtomogram average (transparent grey) as a rigid body. Twenty residues of 96-ES1 (magenta) were not included in the original model and were extended using the tip of a random rRNA ES. ( b ) Zoomed views of the boxed area in a showing colocalization of 96-ES1 and the C1 contact site in more detail. Full size image On the basis of biochemical analyses and knockout experiments, Mba1 was suggested to act as a mitoribosome receptor on the inner membrane and, together with Oxa1, was shown to be required for efficient membrane integration of nascent proteins [7] . Consistent with the proposed function as a mitoribosome receptor, Mba1 fractionates like a bona fide inner membrane protein in flotation gradients ( Supplementary Fig. 6a ) and—upon lysis of membranes with detergents—with mitoribosomes in sedimentation gradients ( Supplementary Fig. 6b ). Moreover, superposition of an atomic model of the mammalian mitochondrial 39S subunit [10] (PDB 4CE4) on the subtomogram average reveals spatial overlap of the modelled fragment of the mammalian Mba1 homologue Mrpl45 and C2 ( Supplementary Fig. 7 ). Taken together, these findings make Mba1 a genuine candidate for mediating the C2 contact. To test this hypothesis, we generated an Mba1 deletion mutant ( Fig. 7a ), which showed defects in the membrane insertion of nascent chains resulting in the accumulation of the precursor form of subunit 2 of cytochrome oxidase ( Fig. 7b ). From this strain, mitochondria were isolated and the in situ structure of the membrane-bound mitoribosome was determined ( Supplementary Fig. 8 ). Consistent with earlier biochemical studies [7] , [8] , the mitoribosome remains tethered to the inner membrane ( Fig. 7c ), likely due to the contribution of 96-ES1 to membrane association of the mitoribosome. Essentially all density assigned to the C2 contact site disappeared, which is also highly significant (>7 s.d.’s) in the difference map to the wild-type structure ( Fig. 7d ). Thus, we identified the second membrane tether of the mitoribosome in the subtomogram average as Mba1 and show where it binds to the mitoribosome to perform its established function as a mitoribosome receptor on the inner membrane. 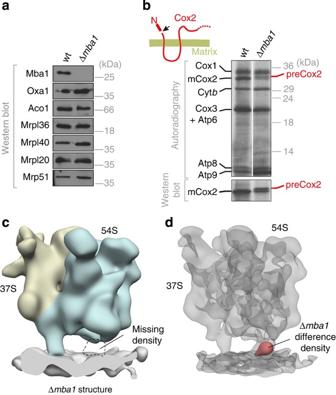Figure 7: The inner membrane protein Mba1 constitutes the C2 contact site. (a) Western blot against the mitochondrial proteins Mba1, Aco1, Oxa1, Mrpl36, Mrpl40, Mrpl20 and Mrp51 in isolated wild-type andΔmba1mitochondria30. Please note that the absence of Mba1 does neither affect the steady-state levels of proteins of the mitoribosome (Mrpl36, Mrpl40, Mrpl20 and Mrp51) nor of the membrane insertase Oxa1. (b) Translation products were radiolabelled for 20 min with [35S]-methionine in isolated wild-type (wt) andΔmba1mitochondria. Synthesized proteins were visualized by SDS–PAGE and autoradiography. The same samples were probed with Cox2-specific antibodies to visualize steady-state levels of endogenous Cox2. Cox2 is initially synthesized in the matrix as a precursor protein (preCox2), which is proteolytically matured after its insertion into the inner membrane by the Imp1 protease in the intermembrane space; mature Cox2 (mCox2) thus depends on the co-translational membrane insertion of Cox2, which is compromised in the absence of Mba1. (c) Subtomogram average of the membrane-bound mitoribosome fromΔmba1mitochondria. Essentially all density assigned to C2 disappeared. (d) Normalized difference density (red) between the structures fromΔmba1and wild-type mitochondria, isosurface-rendered at 7 s.d.’s, superposed to the subtomogram average from wild-type mitochondria (transparent grey). The difference density co-localizes with contact site C2. Figure 7: The inner membrane protein Mba1 constitutes the C2 contact site. ( a ) Western blot against the mitochondrial proteins Mba1, Aco1, Oxa1, Mrpl36, Mrpl40, Mrpl20 and Mrp51 in isolated wild-type and Δmba1 mitochondria [30] . Please note that the absence of Mba1 does neither affect the steady-state levels of proteins of the mitoribosome (Mrpl36, Mrpl40, Mrpl20 and Mrp51) nor of the membrane insertase Oxa1. ( b ) Translation products were radiolabelled for 20 min with [ 35 S]-methionine in isolated wild-type (wt) and Δmba1 mitochondria. Synthesized proteins were visualized by SDS–PAGE and autoradiography. The same samples were probed with Cox2-specific antibodies to visualize steady-state levels of endogenous Cox2. Cox2 is initially synthesized in the matrix as a precursor protein (preCox2), which is proteolytically matured after its insertion into the inner membrane by the Imp1 protease in the intermembrane space; mature Cox2 (mCox2) thus depends on the co-translational membrane insertion of Cox2, which is compromised in the absence of Mba1. ( c ) Subtomogram average of the membrane-bound mitoribosome from Δmba1 mitochondria. Essentially all density assigned to C2 disappeared. ( d ) Normalized difference density (red) between the structures from Δmba1 and wild-type mitochondria, isosurface-rendered at 7 s.d.’s, superposed to the subtomogram average from wild-type mitochondria (transparent grey). The difference density co-localizes with contact site C2. Full size image Mba1 aligns the exit tunnel with membrane-embedded density On the basis of the high-resolution cryo-EM single particle reconstruction of the yeast 54S mitoribosome subunit, the mitoribosomal peptide exit site has been located ~3.5 nm away from the canonical (‘bacterial’) peptide exit, which is blocked by a long mitoribosome-specific extension of Mrpl23 (ref. 9 ). This mitoribosomal peptide channel emerges from the 54S subunit perfectly aligned and face-to-face with Mba1 ( Fig. 8a ), suggesting that Mba1 might be in close contact with nascent peptides emerging from the mitoribosome. Indeed, Mba1 can be chemically crosslinked to nascent but not to mature mitochondrial translation products ( Supplementary Fig. 9 ). In a pull down experiment, immobilized Mba1 can, furthermore, pull down the Oxa1 insertase from mitochondrial extracts, suggesting that Mba1 has the ability to recruit the insertion machinery to the mitoribosome ( Supplementary Fig. 10 ). Indeed, in direct contact with Mba1, an area of particularly high density is discernable inside the inner mitochondrial membrane ( Fig. 8b and Supplementary Fig. 11 ). Thus, in the spatial arrangement observed here, Mba1 may act not only as a passive mitoribosome receptor, but it also may align the membrane-bound mitoribosome with membrane-integral components of the translation machinery, such as the membrane insertion machinery necessary for co-translational protein membrane insertion. 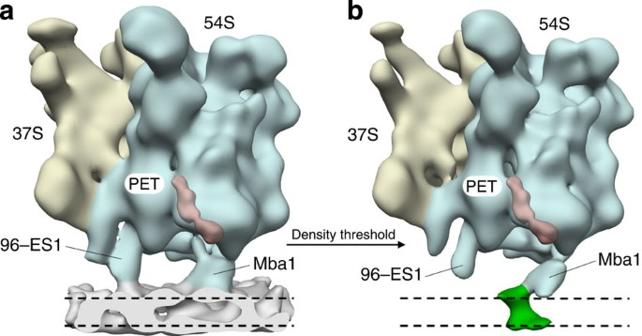Figure 8: Mba1 aligns the ribosomal exit tunnel with a membrane-embedded protein density. (a) Cavity of the peptide exit tunnel (red; PET), as resolved in a single particle reconstruction of the 54S subunit of the yeast mitoribosome9, superposed to the subtomogram average. The peptide exit tunnel emerges from the mitoribosome face-to-face with Mba1. (b) Subtomogram average shown at a higher density threshold level than inato visualize an Mba1-associated, membrane-embedded density (green). Dashed lines indicate the two leaflets of the membrane bilayer. Figure 8: Mba1 aligns the ribosomal exit tunnel with a membrane-embedded protein density. ( a ) Cavity of the peptide exit tunnel (red; PET), as resolved in a single particle reconstruction of the 54S subunit of the yeast mitoribosome [9] , superposed to the subtomogram average. The peptide exit tunnel emerges from the mitoribosome face-to-face with Mba1. ( b ) Subtomogram average shown at a higher density threshold level than in a to visualize an Mba1-associated, membrane-embedded density (green). Dashed lines indicate the two leaflets of the membrane bilayer. Full size image With the help of direct electron detector technology, we could directly visualize mitoribosomes bound to the native inner membrane structures of translation-competent mitochondria in situ , revealing the supramolecular organization of the mitochondrial translation machinery and its association with the inner membrane. Purification and cryopreparation can alter the overall morphology of yeast mitochondria slightly compared with their native counterparts. However, the full functionality in terms of translation and protein membrane insertion ( Fig. 1a ), the structurally well-defined interaction between mitoribosomes and the inner membrane ( Fig. 4 ), and finally the strikingly well-preserved architecture of the delicate polysomal assemblies on the inner membrane ( Fig. 2 ) argue for a mild preparation procedure in our study, preserving the native state of mitochondria with respect to the structural features of its translational machinery. The analysis of mitoribosome arrangements in our study suggests that mitoribosomes are predominantly organized in membrane-bound polyribosomes. The preferred architecture of these polyribosomes is similar to the architecture of polyribosomes bound to the mammalian endoplasmic reticulum [15] . This similarity suggests that the organization of membrane-bound polyribosomes is evolutionarily conserved, probably due to the invariant basic topological requirements for threading an mRNA molecule from one ribosome to next while translocating a nascent peptide across the membrane. Our subtomogram average unveils that the membrane-bound yeast mitoribosome is tethered to the inner mitochondrial membrane by two distinct contacts, one of them the rRNA expansion segment 96-ES1. Involvement of rRNA expansion segments in membrane binding has already been observed for the ER membrane-associated 80S ribosome in situ [15] , suggesting that contribution of rRNA to membrane tethering is a common principle. Whether the negatively charged phosphate residues of the rRNA backbone interact with positively charged head groups of the phospholipids constituting the membrane bilayer, or whether the rRNA specifically interacts with acceptor proteins in the inner mitochondrial membrane, remains to be investigated. The second distinct contact between the mitoribosome and the inner membrane, which is resolved in the subtomogram average, is mediated by the inner membrane protein Mba1. Mba1 is rather ubiquitously found in eukaryotes but absent in bacteria [19] , indicating that this membrane tether might be a general feature of mitoribosomes. In consistence, the mammalian Mba1 homologue Mrpl45 was found in the equivalent position on the mammalian mitoribosome [10] ; however, in that study the position of the membrane remained unclear. In direct contact with Mba1, an area of particularly high density is discernable inside the well-resolved membrane bilayer. The position of this density close to the mitoribosome and its alignment with the peptide exit tunnel suggest that this density could represent a membrane-integral component of the translation machinery, such as the membrane insertion machinery necessary for co-translational protein membrane insertion. The adjacent position of Mba1, together with the multiple reported genetic and biochemical interactions of Mba1 and the Oxa1 insertase, indicate that Mba1 is not simply a passive membrane tether, but rather actively supports mitochondrial protein synthesis by aligning the peptide exit tunnel of the membrane-bound mitoribosome with the membrane insertion machinery. Potentially, Mba1 even supports the transfer of the very hydrophobic mitochondrial translation products towards the membrane insertion machinery to facilitate their fast and reliable insertion ( Fig. 9 ). This would explain the defects in membrane insertion associated with Mba1 deletion ( Fig. 7b ) [7] , [8] . 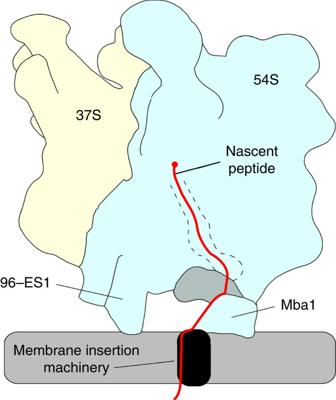Figure 9: Hypothetical model for co-translational membrane protein insertion in yeast mitochondria. The inner membrane protein Mba1 aligns the mitochondrial peptide exit tunnel (dashed lines) with the membrane insertion machinery (black box) and supports the transfer of the very hydrophobic mitochondrial nascent peptides (red line) towards the membrane to facilitate their fast and reliable insertion. Figure 9: Hypothetical model for co-translational membrane protein insertion in yeast mitochondria. The inner membrane protein Mba1 aligns the mitochondrial peptide exit tunnel (dashed lines) with the membrane insertion machinery (black box) and supports the transfer of the very hydrophobic mitochondrial nascent peptides (red line) towards the membrane to facilitate their fast and reliable insertion. Full size image In summary, our analysis of the membrane-bound yeast mitoribosome unveils that, concomitant with the remodelling of the mitoribosomal polypeptide exit tunnel, its membrane association—and potentially also its mode of membrane insertion—have been radically reshaped during evolution. Finally, it demonstrates the power of in situ tomography for the molecular analysis of complex intracellular structures, in particular of those that are as labile as mitochondrial ribosomes. Yeast strains and growth media For imaging of wild-type mitoribosomes, mitochondria were isolated from the wild-type strain D273-10B [20] . Yeast cultures were grown at 30 °C in YP (1% yeast extract, 2% peptone) medium supplemented with 2% galactose [20] . Mitochondria were isolated as described [21] . In brief, for isolation of mitochondria, yeast cells were converted to spheroplasts by incubation with zymolyase (5 mg g −1 wet weight) in 1.2 M sorbitol, 20 mM potassium phosphate for 30 min at 30 °C. Cells were resuspended in homogenization buffer (0.6 M sorbitol, 10 mM Tris-HCl, pH 7.4, 1 mM EDTA, 0.2% (w/v) bovine serum albumin, 1 mM phenylmethylsulphonyl fluoride) and opened in a glass dounce homogenizer. After a clarifying spin for 5 min at 5,000 g , mitochondria were pelleted by centrifugation for 12 min at 12,000 g at 4 °C and resuspended in 0.6 M sorbitol, 20 mM HEPES, pH 7.4 at a protein concentration of 10 mg ml −1 . In organello translation experiments Translation products were labelled in mitochondria as described [21] , [22] . In brief, mitochondria (40 μg protein) were incubated in translation buffer (0.6 M sorbitol, 150 mM KCl, 15 mM KH 2 PO 4 , 13 mM MgSO 4 , 0.15 mg ml −1 of all amino acids except methionine, 4 mM ATP, 0.5 mM GTP, 5 mM α-ketoglutarate, 5 mM phosphoenolpyruvate, 3 mg ml −1 fatty acid-free bovine serum albumin, 20 mM Tris/HCl pH 7.4) containing 0.6 U ml −1 pyruvate kinase and 10 μCi [ 35 S]-methionine. Samples were incubated for 30 min at 24 °C. Labelling was stopped by addition of 25 mM unlabelled methionine. The samples were further incubated for 5 min to complete synthesis and mitochondria were isolated by centrifugation, washed in 1 ml 0.6 M sorbitol, 20 mM Hepes/HCl, pH 7.4 and lysed in 25 μl sample buffer (2% sodium dodecyl sulfate, 10% glycerol, 2.5% β-mercaptoethanol, 0.02% bromophenolblue, 60 mM Tris/HCl pH 6.8). Samples were shaken at 4 °C for 10 min before loading on the gel. Western blotting Western blotting was performed according to the standard protocols. Full scans of all cropped western blots are shown in Supplementary Figs 12–17 . All antisera were raised in rabbits. The antibody against Mrp51 was a kind gift from Tom Fox and the sera against Tim50 was a kind gift from Dejana Mokranjac. Working dilutions of all antibodies are listed in Supplementary Table 1 . Flotation of Mba1 with mitochondrial vesicles Mitochondria (250 μg) were resuspended in 250 mM KCl, 5 mM EDTA, 1 mM phenylmethylsulphonyl fluoride (PMSF), 20 mM Hepes/KOH, pH 7.4 and ruptured by repeated freeze-thawing. One half of the sample was directly applied to SDS–PAGE (total), the other was adjusted to 1.6 M sucrose (300 μl), placed into a centrifugation tube and overlayed with layers of 250-μl 1.2 M sucrose and 100-μl 0.2 M sucrose. The samples were centrifuged in a Beckman SW60 rotor for 16 h at 230,000 g at 4 °C. The gradient was split into a top and bottom fraction and proteins contained were precipitated by addition of trichloroacetic acid (TCA). Aconitase and Oxa1 served as controls for soluble and membrane-embedded proteins, respectively. Sedimentation of Mba1 with mitoribosomes Mitochondria (250 μg) were lysed in 400 μl 1% Triton X-100, 50 mM KCl, 1 mM PMSF, 20 mM Hepes/KOH, pH 7.4. After a clarifying spin for 15 min at 18,000 g at 4 °C, the extract was loaded on a sucrose cushion (100-μl 1.2 M sucrose in lysis buffer) and centrifuged for 1 h at 214,000 g at 4 °C. The supernatant was collected and proteins were prepared by TCA precipitation. Proteins from the pellet (containing mitochondrial ribosomes) were directly dissolved in sample buffer. A total sample containing a comparable amount of mitochondria dissolved in sample buffer was loaded for control. Pull down of Oxa1 with immobilized Mba1 fusion protein Maltose-binding protein (MBP) or an MBP-Mba1 fusion protein [7] was immobilized on amylose beads. Mitochondria (500 μg) were lysed with 1% Triton X-100, 50 mM KCl, 20 mM Hepes/KOH, pH 7.4. The extract was cleared by centrifugation and either directly subjected to SDS–PAGE (4%) or incubated with the MBP proteins as indicated (equivalents to 40%). Proteins were transferred to nitrocellulose and either stained by Ponceau S (lower panel) or probed with Oxa1-specific antibodies. Cryoelectron tomography Translation-competent mitochondria (2 μl) were applied to lacey carbon molybdenum grids (Ted Pella, USA) and incubated for 60 s at 22 °C. Directly before vitrification of the sample in liquid ethane using a Vitrobot Mark IV (FEI, the Netherlands), 4 μl of 10 nm colloidal gold in tomography buffer (20 mM Hepes pH 7.6, 50 mM KCl, 2 mM MgCl 2 ) were added to the grid. Tilt series were acquired using a FEI Titan Krios TEM equipped with a ‘K2 summit’ direct electron detector (Gatan, USA), operated in frame mode with five to seven frames per projection image. The TEM was operated at an acceleration voltage of 300 kV. Single-axis tilt series were recorded from −60° to +60° with an angular increment of 2° at a nominal defocus of 4–8 μm and an object pixel size of 2.62 Å using the Serial EM acquisition software [23] . The cumulative electron dose was 100–120 electrons Å −2 . Image processing Frames from the K2 DDD were aligned using a quasi-expectation maximization protocol implemented in the MATLAB toolbox AV3 (ref. 24 ). Correction of phase reversals due to the contrast transfer function was performed using MATLAB scripts on single projections, as described in ref. 25 . Tomogram reconstruction (object pixel: 2.1 nm) and template matching against a single particle cryo-EM reconstruction of the 73S yeast mitoribosome [9] filtered to 5 nm resolution were accomplished using PyTom [26] . Different rotations of the template were sampled with an angular increment of 12.85°. Tomogram areas corresponding to cross-correlation peaks within mitochondria (distance of distinct peaks >18.9 nm) were visually inspected to identify true-positive matches. For the retained coordinates, unbinned subtomograms (200 3 voxels, object pixel: 0.262 nm) were reconstructed individually from the weighted projections and iteratively aligned using PyTom [26] . Before each iteration, the average was filtered according to its resolution. The optimal translations and rotations of the subtomograms were determined using the constrained correlation function; this similarity measure constrains the correlation between two volumes to their commonly sampled segments in Fourier space. In a first round of Constrained Principal Component Analysis [27] focused on the 37S subunit, 73S mitoribosomes could be separated from remaining false-positives, which could not be excluded by visual inspection, 54S ribosomal subunits and 73S mitoribosomes with a hyper-rotated 37S subunit. In a second round of Constrained Principal Component Analysis focused on the 54S subunit and the membrane region, subtomograms depicting mitoribosomes with clearly visible density for the inner mitochondrial membrane were enriched. The resolution of the resulting averages was determined by Fourier shell correlation (FSC=0.5) and cross resolution (FSC=0.33) with the single particle reconstruction of the 73S yeast mitoribosome [9] on appropriately masked averages. Local resolution estimation was performed using the Bsoft software package [28] . Normalized density difference maps were generated from normalized subtomogram averages, filtered to their respective resolution. The analysis of polyribosome arrangements was carried out in a coordinate system with the z -axis perpendicular to the inner mitochondrial membrane using the full data set of 900 classified mitoribosomes. First, a Gaussian distribution was fitted to the radial pair distribution function of all mitoribosomes in a radius of 100 nm. Only ribosomes within three s.d.’s around the mean distance were used for further analysis. Next, a Gaussian distribution was fitted to the distribution of membrane inclination angles θ in the retained mitoribosome pairs and only mitoribosomes within one s.d. of the mean value were used for further analysis. For each ribosome, we calculated the angle α , describing the relative position of neighbouring ribosomes, and the angle β , describing the relative orientation of neighbouring ribosomes ( Fig. 2a ). The data set was clustered hierarchically in these two dimensions in MATLAB (Mathworks, USA) using the ‘single’ linkage and ‘distance’ clustering criterion. EM-map analysis and tomogram visualization For EM-map analysis, fitting of atomic models, fitting of EM maps, segmentation and visualization, we used the UCSF Chimera software package [29] . Colouration of the EM-maps was performed either on images in Photoshop (Adobe, USA) by applying coloured layers (‘multiply’ style) to the image or in Chimera on segmented densities. For visualization of a whole tomogram in Fig. 1 and analysis of mitoribosome-membrane distances, mitochondrial membranes and selected ATP synthases were segmented manually in Amira (FEI, USA) and the template density of the mitoribosome was positioned according to the coordinates and orientations determined by template matching. How to cite this article: Pfeffer, S. et al . Organization of the mitochondrial translation machinery studied in situ by cryoelectron tomography. Nat. Commun. 6:6019 doi: 10.1038/ncomms7019 (2015). Accession codes : The subtomogram averages for the membrane-associated mitoribosome and the mitoribosome with a hyper-rotated 37S subunit were deposited in the EMDataBank with accession codes EMD 2826 and EMD 2827 , respectively.